Ptychographic electron microscopy using high-angle dark-field scattering for sub-nanometre resolution imaging Diffractive imaging, in which image-forming optics are replaced by an inverse computation using scattered intensity data, could, in principle, realize wavelength-scale resolution in a transmission electron microscope. However, to date all implementations of this approach have suffered from various experimental restrictions. Here we demonstrate a form of diffractive imaging that unshackles the image formation process from the constraints of electron optics, improving resolution over that of the lens used by a factor of five and showing for the first time that it is possible to recover the complex exit wave (in modulus and phase) at atomic resolution, over an unlimited field of view, using low-energy (30 keV) electrons. Our method, called electron ptychography, has no fundamental experimental boundaries: further development of this proof-of-principle could revolutionize sub-atomic scale transmission imaging. In 1936, only 3 years after its invention, Scherzer showed that transmission electron microscopy (TEM) would not be able to reach wavelength-limited resolution (which is possible in light microscopy), by a disheartening factor of about 100, because round magnetic lenses, constrained by the possible configurations of the focusing magnetic field, inevitably have gross aberrations [1] . In 1947, he was also the first to point out that a non-round lens, composed, say, of a number of quadrupoles or sextupoles, could in principle compensate for aberrations [2] . It took until 1997 for the first non-round aberration-correcting electron lens to be successfully demonstrated [3] . The best resolution so far achieved using these very complex systems is about 0.05 nm (50 pm)—but this is still about 25 times poorer than the theoretical diffraction limit (for a review, see ref. 4 ). Further improvement in lens performance faces ever-decreasing marginal gains, first because of the way higher and higher order aberrations begin to dominate the lens correction process, and second because energy spread in the electron source and instabilities in the power supplies sabotage the extreme requirements for coherent interference; a good lens requires electron wave components separated by tens of microns in the back-focal plane to interfere at the image plane (or in the case of the scanning transmission electron microscope (STEM), at the specimen plane) with picometre path-length precision. A radical solution to the limitations of electron lenses is to remove the objective lens completely and measure diffraction patterns rather than images: provided the correct phase structure can be assigned to this diffraction data, it can then be inverted to realize a completely aberration-free image. There has been much research over the last decade into this diffraction phase problem (a method called coherent diffractive imaging), particularly within the X-ray community [5] , [6] , [7] . If the specimen or region of interest is two-dimensional and of finite extent, then it turns out that there is usually a unique solution to the phase of the diffraction pattern [8] . This is because if the estimate of the phase is wrong, then the Fourier components composing the object will not cancel to zero outside its known dimensions. This technique has been shown to work for electrons [9] , including in the transmission mode in a scanning electron microscope (SEM) [10] , [11] . A hybrid method complementing conventional image data with diffraction data has also been implemented [12] . Holographic, totally lensless methods have also been implemented [13] , [14] , [15] . But all of these techniques can only image an extremely small field of view; practical microscopy must allow for an indefinite field of view, which is achieved by the approach we report here. The theoretical concept of the method we use—ptychography—was first postulated 40 years ago [16] , [17] , [18] , [19] , [20] , [21] . However, practical iterative solution methods for recovering the inverse calculation are relatively recent [22] , [23] , [24] , [25] , [26] , [27] , [28] , [29] , [30] , [31] , [32] . The technique overcomes all the shortcomings of both conventional lens imaging and conventional single exposure coherent diffractive imaging [23] , [25] , [26] , [27] , [28] , [29] , [30] . A localized area of illumination is moved to a number of positions over the object (in our case, around 100–900). If we arrange for the areas of illumination to overlap with one another, redundancy in the recorded data allows for very quick and robust solution of the phase problem [30] : we can solve for the phase of each diffraction pattern in less than a second. We can then back propagate the wave function to the object plane and thus construct an image with a resolution determined only by the effective numerical aperture of the detector: that is, the sine of the angle the detector subtends at the specimen. The concept of ptychography was first demonstrated at atomic wavelengths using 100 keV electrons, but only with a crystalline (silicon) specimen, and was shown to be able to obtain images (albeit of a simple unit cell) at about a factor of three times better resolution than that of the transfer function of the microscope used [33] . Iterative phase-retrieval ptychography allows for the imaging of any type of structure. In addition to the possibility of wavelength-limited resolution, a key property of ptychography is that it recovers the phase of the wave that has travelled through the specimen with great accuracy and with high contrast. This means, for example, that it can be used for the structural discovery of very weakly absorbing specimens; it has been shown to work for three-dimensional (3D) X-ray tomography of low-density biological material [32] . The broad principle of this iterative approach has also recently been demonstrated for high-energy electrons (200 keV), but for the case of processing only the central disk (Ronchigram) of the diffraction pattern in order to calculate the phase of the wave transmitted through the object [34] . The resolution of the image so obtained was therefore limited by the electron optics to 1 nm; about six times larger than the intrinsic conventional resolution of the 200 keV microscope that was used to collect the data. In this paper, we process the dark-field, high-resolution intensity to observe atomic-scale structure using 30-keV electrons in an SEM of standard specification, surpassing the intrinsic resolution of the microscope we use by a factor of about five. Our results are transmission images, not conventional SEM images: we are performing TEM imaging within an SEM without any magnification optics. If we were to use the lens in this system to form a conventional image at this low accelerating voltage, we would expect a best (and optimistic) resolution of 1.2 nm: here we obtain images with about 0.24 nm resolution in both modulus and phase over an indefinitely large field of view. The concept demonstrated here has no ultimate resolution limit, except those determined by the electron wavelength (between about 1/20 and 1/100 of an atomic diameter, depending on the electron energy), specimen damage, and the scattering and vibration properties of the atoms themselves. Description of experimental setup We use a SEM with a thermally assisted Schottky field emission gun (FEG) and the optical setup shown in Fig. 1 for our experiments. Instead of bringing the electrons to focus at the specimen plane, we under-excite the objective lens so that the beam crossover moves down the column by ∼ 3 μm. Consequently, there is a relatively broad patch of illumination (20–40 nm in diameter) incident upon the specimen. Note that the lens can be of low quality (aberrated) because it is not being used to image the specimen; it is rather a means of condensing the electron radiation into an approximately localized region. 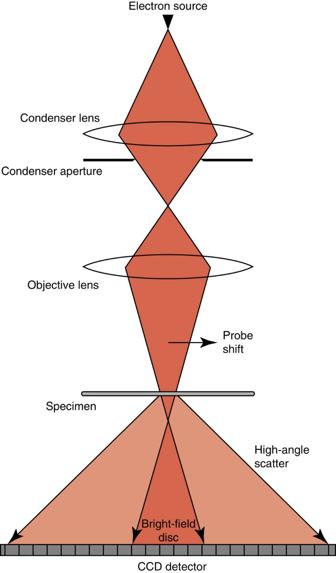Figure 1: Schematic of the experimental arrangement. Experiments were carried out on an FEI Quanta 600 SEM fitted with a thermally assisted Schottky field emission gun and operating at 30 keV. The probe wavefront was formed using the microscope condenser and objective lenses and was scanned across the specimen using the microscope scanning coils. The specimen was mounted on a compact rig attached to the objective lens pole piece assembly. The door of the microscope was replaced in order to accommodate a flange for a Gatan Orius SC200 CDD camera that was cantilevered into a position below the specimen plane. Figure 1: Schematic of the experimental arrangement. Experiments were carried out on an FEI Quanta 600 SEM fitted with a thermally assisted Schottky field emission gun and operating at 30 keV. The probe wavefront was formed using the microscope condenser and objective lenses and was scanned across the specimen using the microscope scanning coils. The specimen was mounted on a compact rig attached to the objective lens pole piece assembly. The door of the microscope was replaced in order to accommodate a flange for a Gatan Orius SC200 CDD camera that was cantilevered into a position below the specimen plane. Full size image The main modification we have made to the microscope is that a CCD detector is positioned at the bottom of the specimen chamber. The CCD records the diffraction pattern, as exemplified by Fig. 2 ; in the centre of the pattern is a bright disk, which is a shadow image cast by the condenser aperture, and which is of the form of a Gabor hologram [35] (otherwise known in the STEM literature as a Ronchigram'). Within this, diffracted amplitude interferes with a relative strong unscattered beam. Outside the central disk, we have so-called dark-field diffracted intensity. 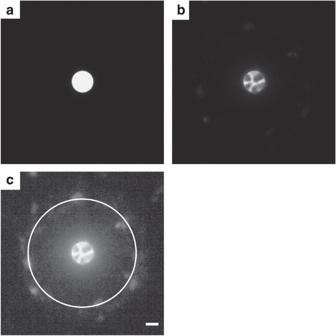Figure 2: Examples of the recorded diffraction patterns. (a) Free-space diffraction pattern, that is, collected when the probe is in free space. The disk is a shadow image cast by the condenser aperture. (b) Diffraction pattern from the sample. The strong bright-field intensity is seen inside the central disk, also known as the Gabor hologram or Ronchigram. (c) The same diffraction pattern as shown inbplotted on a log-intensity scale to show dark-field intensity data: the high-resolution information arises from this data. Scale bar, 1 nm−1. The ring indicates a radius of 0.236 nm−1. Figure 2: Examples of the recorded diffraction patterns. ( a ) Free-space diffraction pattern, that is, collected when the probe is in free space. The disk is a shadow image cast by the condenser aperture. ( b ) Diffraction pattern from the sample. The strong bright-field intensity is seen inside the central disk, also known as the Gabor hologram or Ronchigram. ( c ) The same diffraction pattern as shown in b plotted on a log-intensity scale to show dark-field intensity data: the high-resolution information arises from this data. Scale bar, 1 nm −1 . The ring indicates a radius of 0.236 nm −1 . Full size image By the standards of conventional TEM, we use a very low accelerating voltage (30 keV). For many years, the main strategy for improving TEM resolution was to work at high voltage, thus decreasing the electron wavelength. A typical medium performance TEM (no aberration correction) working at 200 keV can routinely achieve just under a 0.2-nm resolution. However, at these energies, the electrons have sufficient momentum to displace atoms into interstitial sites or completely out of the specimen, creating 'knock-on' damage. For the lightest elements, such as carbon, atoms can be displaced with an electron energy of only 50 keV (ref. 36 ). An advantage of low electron energy, which we exploit here, is that the cross-section of interaction with the atomic potential increases, so that the diffraction pattern has good signal-to-noise ratio at high-scattering angles (high-resolution data is more strongly expressed). However, for weakly bound soft matter, such as biological samples where the dominant damage mechanism is radiolysis or heating, it is advantageous to work at high voltage. Ptychography can work at any accelerating voltage, and so in practice one would choose to operate at a point where competing damage mechanisms add up to an overall minimum. As an aside, it should be pointed out that the cross-section of scattering for X-rays is about four orders of magnitude smaller than that of electrons, and so only electrons can offer practical sub-atomic resolution. Despite the fact that the wavelength of a 30-keV electron is about 2.8 times larger than that of a 200-keV electron, the image resolution we obtain here is comparable to that of a 200-keV microscope. These figures are quite extraordinary, given that the SEM we use in transmission mode is not optimized for atomic-scale experiments—its stability envelope is designed for 1–2 nm scale secondary electron imaging. The key to our approach lies in the fact that intensity residing in the dark-field area of the detector relates to very-high-frequency components in the specimen. A conventional STEM operated in either conventional bright-field or dark-field mode relies for its resolution on the narrowness of the beam crossover, which itself is determined by the diameter of the central disk, that is, the solid angle embraced by the lens (see Fig. 2 ). However, by processing the dark-field data and inverting it into an image, we can in principle obtain resolution inversely proportional to the scattering angle captured by the detector (tens of degrees), which is many times larger than the useable lens transfer function (typically one or two degrees). The problem we face is that in order to calculate the structure of the object we must compute the phase of the high-angle diffracted intensity, so that the high-frequency (Fourier) components of its image can be assembled correctly. Details of reconstructed images We use the extended ptychographical iterative engine (ePIE) to re-phase the recorded diffraction data and reconstruct our images [30] . 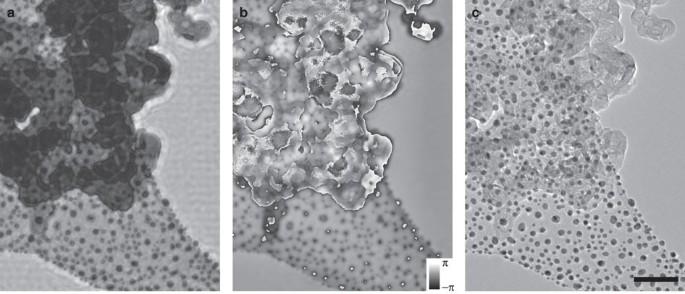Figure 3: Wide-field ptychographic reconstruction of gold particles and graphitized carbon on a holey carbon support film. (a) Modulus and (b) phase of the ptychographic reconstruction. (c) Comparison with the conventional TEM image of the same area taken at 200 keV. Note the strong contrast ina, and thatbexhibits phase wraps in thick areas of the object, that is, the phase passes from π to −π, forming a contour-like plot of thickness. Scale bar, 50 nm. Figure 3 shows the reconstructed modulus and phase image of a standard TEM test specimen consisting of a holey carbon film scattered with dispersed gold particles approximately ranging from 2 to 5 nm in diameter, and also relatively thick clumps of graphitized carbon. In the conventional TEM micrograph, the bright-field image has very low contrast and, because of the transfer properties of the lens, does not express accurately the phase of the exit wave. With ptychography, we see the absolute phase induced into the transmitted electron wave over the entire field of view, a signal that is directly proportional to the product of the thickness of the specimen and its inner potential. Figure 3: Wide-field ptychographic reconstruction of gold particles and graphitized carbon on a holey carbon support film. ( a ) Modulus and ( b ) phase of the ptychographic reconstruction. ( c ) Comparison with the conventional TEM image of the same area taken at 200 keV. Note the strong contrast in a , and that b exhibits phase wraps in thick areas of the object, that is, the phase passes from π to −π, forming a contour-like plot of thickness. Scale bar, 50 nm. Full size image The thickness of the layer of graphitized carbon at the top of the specimen has introduced phase wraps and phase vortices into Fig. 3b , and has resulted in a Fresnel-type fringe at the interface between the edge of the carbon and free space, an effect that has also been observed in ptychography at X-ray wavelengths [37] . These features indicate that the thickness of the specimen here is approaching the limit of validity of the projection approximation upon which our reconstruction algorithm relies. Specimen thickness also impacts upon the interpretable resolution of the image, because of the curvature of the Ewald sphere in reciprocal space. It has been shown that it is possible to extract an actual high-resolution projection of a thick object from the ptychographic data set [38] , and that this can in principle be extended to obtaining multiple projections of the object [39] . However, this approach is not very practical because it relies upon the specimen being weakly scattering and requires the illumination to be moved over a grid of positions corresponding to the pixel resolution of the final reconstruction. We are optimistic that we can account for these 3D scattering effects in the framework of an iterative method similar to the ePIE, however, this work is still at an early stage. 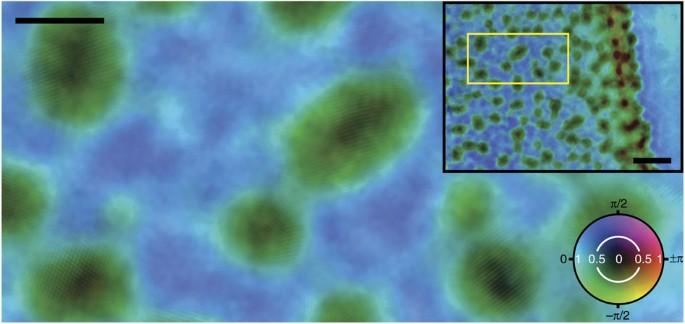Figure 4: Ptychographic reconstruction of gold particles showing the atomic fringes. The full field-of-view is shown in the inset image (scale bar, 15 nm); the main image is a blow up of the region indicated by the yellow box, showing 0.236 nm atomic plane fringes (scale bar, 5 nm). The modulus and phase of the reconstructions are combined in these images, with phase represented by colour and modulus by brightness, as indicated on the colour wheel scale. Figure 4 shows a magnified image of several of the gold particles in a thin area of the object where the thickness issues described above do not apply. The <111> atomic planes are clearly visible in some of the particles: the spacing we measure from the image is 0.24 nm, compared with the expected value of 0.236 nm. Note that the calibration of the image magnification follows directly from the measured electron wavelength, the camera length and the dimensions of the CCD. The fringes do not occur in all the particles, and usually not over the whole of any one particle (which are known to be multiply-twinned), because for many crystalline orientations the projected planes cannot be resolved. In conventional bright-field coherent TEM imaging, the exact location of fringes associated with a particular set of Bragg planes can often be delocalized from their true real-space position. As the objective lens is defocused, periodic features are seen to cross over one another. In ptychography, the correct defocus should be guaranteed because, for a given probe shift, there is only one reconstruction focus which is consistent with the measured data, at least for the thin area of specimen examined here. In theory, the computational transfer function of the technique is perfect, so our images preserve all Fourier components, including the low frequencies that are lost in TEM. Figure 4: Ptychographic reconstruction of gold particles showing the atomic fringes. The full field-of-view is shown in the inset image (scale bar, 15 nm); the main image is a blow up of the region indicated by the yellow box, showing 0.236 nm atomic plane fringes (scale bar, 5 nm). The modulus and phase of the reconstructions are combined in these images, with phase represented by colour and modulus by brightness, as indicated on the colour wheel scale. Full size image Our phase-retrieval algorithm also reconstructs the structure of the illuminating electron beam incident upon the sample during data collection. For the results shown in Fig. 4 , the recovered illumination function is shown in Fig. 5 , together with its Fourier transform (that is, the form of the condenser aperture), which can be compared directly with Fig. 2a . By propagating this wavefront, the profile shown in Fig. 6 of the illumination along the optical ( z ) axis of the microscope, can also be derived. As these results are exactly consistent with what we expect, we are confident that the reconstruction is also self-consistent and accurate. Specifically, this implies that specimen thickness, partial coherence and inelastic scattering (see below) have not significantly affected the reconstruction. However, we should nevertheless interpret the results with some caution; as in a conventional TEM operated at this low accelerating voltage, multiple scattering must also affect our images to some extent, even though the thickness of the particles is <5 nm. 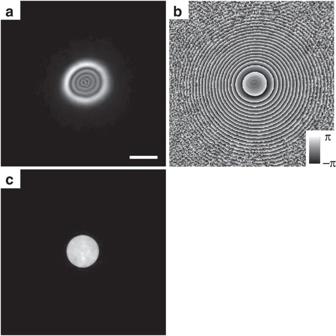Figure 5: Example of a reconstructed probe wavefront. Modulus (a) and phase (b) of the probe as derived via the ePIE. (c) Modulus of the Fourier transform of the probe, which compares accurately to the recorded free-space diffraction pattern. These functions are exactly as we would expect them to be. Although the real-space probe cannot be imaged in SEM, the ring structure and slight astigmatism is commonly seen in TEM. The round condenser aperture (which again cannot be measured directly in SEM) implies the phase and modulus of the real-space probe is consistent with the physical electron optics. Figure 5: Example of a reconstructed probe wavefront. Modulus ( a ) and phase ( b ) of the probe as derived via the ePIE. ( c ) Modulus of the Fourier transform of the probe, which compares accurately to the recorded free-space diffraction pattern. These functions are exactly as we would expect them to be. Although the real-space probe cannot be imaged in SEM, the ring structure and slight astigmatism is commonly seen in TEM. The round condenser aperture (which again cannot be measured directly in SEM) implies the phase and modulus of the real-space probe is consistent with the physical electron optics. 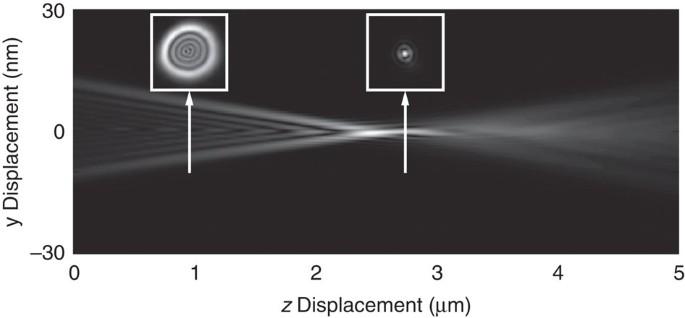Figure 6: Transverse profile of the probe modulus along the optic axis of the microscope. The plot was calculated by forward and back propagating the complex stationary wave of the probe function that is derived by the phase-retrieval algorithm. The pronounced spherical aberration present in the beam is apparent from this plot. The insets plot thex–yprofile of the probe at thezpositions indicated by the white arrows, on the scale indicated on theyaxis. The left-hand inset plots the probe at the plane of the specimen and the right-hand inset plots the probe propagated to the focus of the beam. Full size image Figure 6: Transverse profile of the probe modulus along the optic axis of the microscope. The plot was calculated by forward and back propagating the complex stationary wave of the probe function that is derived by the phase-retrieval algorithm. The pronounced spherical aberration present in the beam is apparent from this plot. The insets plot the x–y profile of the probe at the z positions indicated by the white arrows, on the scale indicated on the y axis. The left-hand inset plots the probe at the plane of the specimen and the right-hand inset plots the probe propagated to the focus of the beam. Full size image We have demonstrated for the first time that electron ptychography can overcome the lens-defined resolution limit in TEM over an unlimited field of view. The phase and modulus transfer function of the technique in theory is perfect, unlike conventional bright-field imaging, where the phase transfer function is uneven, has zeros, and loses the low-frequency information entirely, thus leading to significant image artefacts. Previous work in iterative phase-retrieval electron ptychography has not used the high-angle dark-field diffraction intensity, and so has not been able to improve on the intrinsic resolution of the lens used to form the region of illumination at the specimen [34] . Unlike conventional forms of electron diffractive imaging, which require knowledge of the size of an isolated object or the form of a localized illuminating beam [8] , [9] , [40] , ptychography can handle any field of view or any form of unknown structured illumination. Apart from resolution improvement, we believe that the quantitative properties of the ptychographic phase image will also have many applications: for example, imaging of magnetic domains, mapping of magnetic and electric fields, and the measurement of inner potentials. Indeed, all applications of electron holography could be undertaken by ptychography—but with the added advantages of high resolution, much lower requirements on the stability and coherence of the experimental setup, wider field of view, and no need for an area of free space adjacent to the area of interest. The main sources of error in our approach arise from inaccuracies in the position of the illumination (hysteresis occurs in the microscope shift coils), the calibration of the camera length (the specimen–detector distance), calibration of the illumination shift step size and the noise floor and read-out properties of the CCD camera. General mechanical and electrical instabilities in the microscope column must clearly affect the effective degree of spatial coherence in the entire setup, which we know reduces the resolution of the technique. The principal source of partial coherence is the angular size of the illumination source (the 'spot size') subtended at the back-focal plane of the probe-forming lens, yet experiments over a range of spot sizes show very little degradation in the quality of the reconstructed images. This is in part attributable to our use of a defocussed probe, which is known to reduce the required degree of coherence in diffractive imaging [41] . Ultimately, the resolution limit for ptychography will in part be determined by the practicality of preparing very thin specimens to avoid 3D scattering effects or, as discussed above, by our ability to account for these effects during the reconstruction process. It will also be affected by two further issues. The first is specimen damage, which will increase as the radiation per unit area is necessarily increased to realize higher resolution. A possible advantage of ptychography in this respect is that the phase image has high contrast. The second is that inelastic scattering may mask the coherent scattering we rely upon for this technique to work. Exactly how serious this will be is uncertain: it has not affected the results we present here, where no attempt has been made to energy filter the scattered electrons, but clearly further work is required in this area. It should be emphasized that current results represent a first step in what we believe is a completely new epoch of electron imaging. Many improvements in the experimental setup can be envisaged. The resolution that we achieve here is determined by the angle that the detector subtends at the specimen—a simple, non-fundamental, geometric constraint. Combining an optimal detector configuration with reduced wavelength (by working at normal TEM accelerating voltages: 80–300 keV) could in principle let us achieve much less than 0.05 nm resolution: better than the very best state-of-the-art aberration-corrected machines. Although here we have used a conventional round magnetic lens to form the illumination at the object plane, there are undoubtedly much better ways to configure and optimize a ptychographic microscope. The only requirement on the illumination is that it is reasonably localized (say up to 100 times larger than the final resolution desired) and coherent. There is no need for a high-performance objective lens or any magnification optics. By disposing of so many high-precision components, and moving the imaging process into a computer, we can at last see a route to exploiting the shortness of the electron wavelength for ultimate transmission imaging. No longer does TEM have to be bound by the paradigm of the lens—its Achilles' heel since its invention in 1933. Experimental method The SEM used in these experiments was an FEI Quanta 600 FEG fitted with a thermally assisted Schottky FEG. Its nominal resolution for the backscattered image, as quoted by the manufacturer, is 2.5 nm. The nominal resolution of the secondary electron image when working at 30 keV (as here) is 1.2 nm. The door of the microscope was replaced in order to accommodate a flange for a Gatan Orius SC200 CDD camera (with a 14-bit dynamic range and 2,048×2,048 pixels on a 7.4-μm pitch), which was cantilevered into a position below the specimen plane. The manufacturer's specimen stage was replaced by a compact rig attached to the objective lens pole piece assembly: this was to minimize specimen vibration and drift. Drift rates for the experiments reported here were of the order of about 1 nm min −1 . A simple manual positioning mechanism built into the rig enabled displacement of the specimen to select the field of view. In any one field of view, the shift of the illuminating beam required for collecting ptychographical diffraction patterns was achieved with the microscope scan coils. The angle of convergence of the probe-forming optics was calibrated using diffraction patterns obtained from crystalline silicon. We note that this angle is not a simple linear function of condenser and/or objective excitation or working distance, and hence, had to be tabulated for the range of lens settings used. The camera length (that is, the distance between the specimen and the detector) was measured directly and found to be 12.7 cm. To reduce the influence of contamination, the chamber was plasma cleaned for 1 h before experimental runs. The readout of the CCD camera was programmed to minimize the duty cycle. Typical exposure times were about 60 ms. In its normal configuration, the readout and file-write time of the system we used is usually about 1 s. This was reduced to 100 ms by low-level programming of the read-out routines and by storing all data from any one experiment into RAM, before saving to the disk. Ptychography requires the object to be illuminated by a patch of radiation—the probe function. In the absence of specimen drift or other time-dependent changes, it is advantageous to have this be as large as possible, so that a wide field-of-view can be examined with only a few probe positions. The maximum size of the illumination area is determined by the need to fulfil the angular Nyquist sampling condition in the diffraction plane. For the configuration described here, this size is fixed by the camera pixel size and the camera length at a maximum of 40 nm; if 2×2 pixel binning is activated on the camera, this reduces to 20 nm. The probe radius can be estimated geometrically by forming the product of defocus times the convergence semi-angle of the beam, but this is very approximate. We relied on the ePIE reconstruction (see below) to give an estimate of the probe function and used this as a check on the actual probe size. In the results presented in Fig. 3 , the probe diameter was 40 nm, the probe step size was 10 nm, and it was scanned over an array of 31×31 positions with an overlap parameter of 75%. The entire data set of 961 patterns took 190 s to collect. The average integrated counts per diffraction pattern was 4×10 7 electrons. The probe positions used were on a substantially rectilinear grid, but known random offsets were introduced of about 25% of the overlap in order to suppress periodic artefacts in the reconstruction. In the results presented in Fig. 4 , the diffraction patterns were binned and the probe diameter was 20 nm. The probe step size was 5 nm, and it was scanned over an array of 20×20 positions, with an overlap parameter of 75%. Image reconstruction procedure Image reconstruction followed the iterative method described by Maiden and Rodenburg [30] , which we call ePIE, summarized briefly in the following. The iterative solution starts by assuming that the complex-valued object transmission function is unity over the two-dimensional plane of the specimen, that is, O ( x , y )=1. A rough estimate of the probe function P ( x , y ) is also required and is generated based on the amount of defocus described above. We label the intensity of the diffraction patterns by I j ( u , v ), where u and v are coordinates describing the detector plane and the patterns are indexed by j =1,2...J . The x and y lateral displacements of the probe when the j th pattern was collected are labelled X j and Y j , respectively. Beginning with a randomly selected value of j , we form a current guess of the exit wave function emanating from the specimen according to: and then form its Fourier transform Ψ g ( u , v ). The modulus of Ψ g ( u , v ) is replaced with , but its phase is preserved to give Ψ c ( u , v ), a corrected guess of the far-field diffracted wave. Ψ c ( u , v ) is inverse Fourier transformed to give a corrected guess of the exit wave field ψ c ( x , y ). An updated estimate of the object function is next computed according to: where max denotes the maximum value of a function, and * denotes the complex conjugate. In the work reported here, we use α =1, although other values of α can be beneficial in accelerating or slowing convergence of the algorithm. An updated estimate of the probe function is formed in a similar manner: where again β =1 was used in the presented results, but can be varied to control convergence of the algorithm. Repeating the above steps for each j completes a single iteration of the ePIE. Iterations continue until a terminating condition is met, or until a fixed number of iterations have been completed. For more details of convergence properties, see ref. 30 . How to cite this article: Humphry, M.J. et al . Ptychographic electron microscopy using high-angle dark-field scattering for sub-nanometre resolution imaging. Nat. Commun. 3:730 doi: 10.1038/ncomms1733 (2012).